AmotL2 disrupts apical–basal cell polarity and promotes tumour invasion The establishment and maintenance of apical–basal cell polarity is essential for the functionality of glandular epithelia. Cell polarity is often lost in advanced tumours correlating with acquisition of invasive and malignant properties. Despite extensive knowledge regarding the formation and maintenance of polarity, the mechanisms that deregulate polarity in metastasizing cells remain to be fully characterized. Here we show that AmotL2 expression correlates with loss of tissue architecture in tumours from human breast and colon cancer patients. We further show that hypoxic stress results in activation of c-Fos-dependent expression of AmotL2 leading to loss of polarity. c-Fos/hypoxia-induced p60 AmotL2 interacts with the Crb3 and Par3 polarity complexes retaining them in large vesicles and preventing them from reaching the apical membrane. The resulting loss of polarity potentiates the response to invasive cues in vitro and in vivo in mice. These data provide a molecular mechanism how hypoxic stress deregulates cell polarity during tumour progression. The formation of three-dimensional (3D) epithelial structures in organs such as the breast, prostate and colon is dependent on the establishment of cell polarity. This general term describes the asymmetrical distribution of molecules and organelles within a cell, and is exemplified by molecular segregation observed in budding yeast, neuronal signalling and migrating cells [1] , [2] . Without this molecular segregation and cellular organization, specialized function is often lost. For example, breast epithelia will only produce milk in an environment that supports apical–basal polarization [3] . The establishment and the maintenance of apical–basal cell polarity and eventually the depolarization of a cell is a complex process controlled by a set of core protein complexes. These include the Par3/Par6/aPKC and Crumbs/Pals1/PATJ proteins that define the apical membrane and Scribble/Lgl/Dlg that promote baso-lateral membrane formation [4] . The evolutionary conserved proteins localize asymmetrically before morphological polarization and mutually antagonize each other [5] . The maintenance of cell polarity is a highly dynamic process as interference with vesicle trafficking proteins such as Rab8 and Rab11 results in loss of already established cellular asymmetry [6] , [7] , [8] . The majority of human cancers arise in tissues of epithelial origin and account for >80% of all cancer-related deaths ( http://www.cancer.org/ ). A strong correlation between malignancy and loss of epithelial organization has been documented for most carcinomas that may be attributed to loss of polarity [9] . The deregulation of apical–basal polarity is often depicted as a hallmark of cancer, although direct evidence, whether this is a cause or consequence of tumour progression, is not yet clear [10] , [11] . Evidence for a growth-suppressive role of cell polarity stems from findings in Drosophila in which the polarity proteins such as Crumbs, Scribble, Dlg and Lgl act as tumour suppressor genes [9] . Furthermore, recent work point to the existence of a similar role in mammalian cells as loss of expression of either Crumbs/Crb3 or Scribble promotes tumour progression in mouse tumour model systems [12] , [13] . In human breast cancer, loss of Par3 expression is associated with a higher tumour grade and ErbB2-positive status. Depletion of Par3 in experimental settings was also associated with increased MMP9 expression and E-cadherin dynamics contributing to an invasive phenotype [14] . It is thus becoming increasingly clear that the deregulation of the polarity proteins is an intrinsic part of tumour progression. AmotL2 belongs to the Angiomotin (Amot) family of membrane-associated scaffold proteins and contains an amino-terminal glutamine-rich domain, coiled-coil repeats and a carboxy-terminal PDZ (for Psd-95 (postsynaptic protein), DlgA ( Drosophila disc large tumour suppressor) and ZO1 (zona occludens))-binding domain that together structurally define the Amot family [15] . We have previously shown that each member has a distinct role in blood vessel formation in that Amot controls migration, AmotL1 junction formation and AmotL2 aortic lumen expansion [16] , [17] , [18] . Acting as a scaffold protein, AmotL2 and its related proteins associate and join together proteins involved in junction formation, apical polarity and actin cytoskeleton [19] . It is therefore conceivable that one of the main functions of the Amot family is to integrate these signalling pathways to regulate cellular shape. Of particular interest are the recent findings that Amot proteins are involved in the control of the HIPPO pathway. Amot proteins associate with the HIPPO effector Yap1 and negatively regulate its activity by sequestration in the cytoplasm (detailed review can be found in ref. 20 ). Hypoxia is a characteristic feature of locally advanced tumours and is coupled to tumour invasiveness, poor survival and treatment failure in cancer patients [21] . The cellular adaptation to hypoxia may also contribute to loss of polarity, tissue integrity and architecture. However, little is known regarding the molecular mechanisms by which a hypoxic environment influences polarity. Here we show that hypoxia-induced p60 AmotL2 is a central component in the negative regulation of tumour cell polarity and may contribute to metastatic spread. AmotL2 expression in breast and colon cancer The reported regulation of AmotL2 by hypoxia and its effect on cellular migration prompted us to analyse the expression pattern of AmotL2 in human cancer [15] , [22] , [23] , [24] . AmotL2 protein expression was detected by immunohistochemical staining of paraffin-embedded sections from breast and colon cancer patients. Normal breast epithelia were negative for AmotL2 but showed positive staining for the apical membrane marker Crb3 ( Supplementary Fig. 1 ). Polarized glandular tumours were AmotL2 negative, whereas depolarized tumour cells growing within mammary ducts were positive for AmotL2 (ductal carcinoma in situ ; Fig. 1a,b,d–f and Supplementary Fig. 1 ). Tumour cells infiltrating the surrounding stroma also showed strong positivity for AmotL2 ( Fig. 1c,g ). Of interest was that positive signal was confined to intracellular large vesicles ( Fig. 1f,g ). 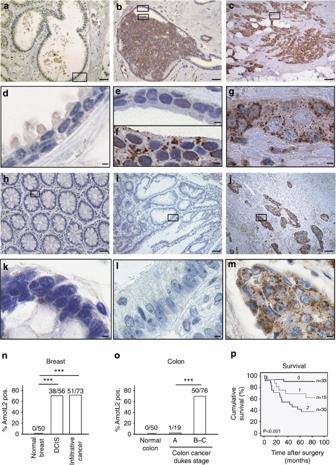Figure 1: AmotL2 expression in human breast and colon cancer correlates with loss of polarity. Analysis of AmotL2 expression in human breast and colon cancer samples was analysed by immunohistochemical staining of paraffin sections. (a,d) AmotL2 expression was not detectable in hyperplastic mammary polarized tumours. (b,e,f) AmotL2 positivity (pos.) in ductal carcinomain situ(DCIS), note that the polarized normal epithelium of the duct is negative. (c,g). AmotL2 was also positive in infiltrative ductal carcinoma. (h–m) AmotL2 expression was analysed in colon cancer samples from Dukes grade A–C. No expression of AmotL2 could be detected in normal colon (h,k). Central polarized areas of Dukes C tumours were also negative (i,l), whereas budding cells of the invasive front were positive (j,m). (n) Summary of AmotL2 positivity in normal breast, DCIS and invasive breast cancer. Normal breastn=50, DCISn=56, infiltrative cancern=73. (o) Summary of AmotL2 immunostainings of colon cancer tissues. Normal colonn=50, colon cancer Dukes An=19, colon cancer Dukes B–Cn=76, ***P≤0.001 as calculated by theχ2-test. (p) AmotL2 expression was correlated in Kaplan–Meier plots to overall survival. Immunohistochemical staining intensity was defined by a visual grading scale 0–2 based on intensity as well as its focal extent (grade 0=no staining, grade 1<25% positivity and grade 2>25% positivity).Pvalues from pairedt-tests, ***P<0.001. Scale bars, 80 μm (a–c,h–j) and 5 μm (d–g,k–m). Figure 1: AmotL2 expression in human breast and colon cancer correlates with loss of polarity. Analysis of AmotL2 expression in human breast and colon cancer samples was analysed by immunohistochemical staining of paraffin sections. ( a , d ) AmotL2 expression was not detectable in hyperplastic mammary polarized tumours. ( b , e , f ) AmotL2 positivity (pos.) in ductal carcinoma in situ (DCIS), note that the polarized normal epithelium of the duct is negative. ( c , g ). AmotL2 was also positive in infiltrative ductal carcinoma. ( h – m ) AmotL2 expression was analysed in colon cancer samples from Dukes grade A–C. No expression of AmotL2 could be detected in normal colon ( h , k ). Central polarized areas of Dukes C tumours were also negative ( i , l ), whereas budding cells of the invasive front were positive ( j , m ). ( n ) Summary of AmotL2 positivity in normal breast, DCIS and invasive breast cancer. Normal breast n =50, DCIS n =56, infiltrative cancer n =73. ( o ) Summary of AmotL2 immunostainings of colon cancer tissues. Normal colon n =50, colon cancer Dukes A n =19, colon cancer Dukes B–C n =76, *** P ≤0.001 as calculated by the χ 2 -test. ( p ) AmotL2 expression was correlated in Kaplan–Meier plots to overall survival. Immunohistochemical staining intensity was defined by a visual grading scale 0–2 based on intensity as well as its focal extent (grade 0=no staining, grade 1<25% positivity and grade 2>25% positivity). P values from paired t -tests, *** P <0.001. Scale bars, 80 μm ( a – c , h – j ) and 5 μm ( d – g , k – m ). Full size image The expression pattern of AmotL2 was also analysed in specimen from colon cancers with local invasion classified according to Dukes stage (Dukes A, tumours confined to the mucosa and sub-mucosa, and Dukes B–C confined to tumours penetrating the muscle wall). Similar to breast tissues, AmotL2 was not detected in normal colon epithelia ( Fig. 1h,k ). The polarized villous structures in the center of the tumours were characteristically AmotL2 negative ( Fig. 1i,l ), whereas the budding cells in the tumour front were AmotL2 positive ( Fig. 1j,m ). Similar to breast cancer, AmotL2-positive staining localized to intracellular large vesicles ( Fig. 1m ). Approximately 65% of all breast ( Fig. 1n ) and Dukes B-C colon tumours ( Fig. 1o ) were positive for AmotL2. Approximately 65% of the Dukes B–C patients showed positive staining for AmotL2 in the invasive front ( Fig. 1o ). Kaplan–Meier analysis of AmotL2 expression and patient survival data showed that AmotL2 is a marker of poor prognosis in colon cancer ( Fig. 1p ). Human AmotL2 encodes two isoforms of a molecular mass of 100 kDa (gene accession no. Q9Y2J4) and 60 kDa (gene accession no. AAH11454; ref. 15 ). Both breast and colon tumour tissues were negative for immunohistochemical staining using a p100 AmotL2-specific antibody ( Supplementary Fig. 1 ). Taken together, these data indicate a correlation between p60 AmotL2-positive vesicular structures and malignancy. c-Fos activates p60AmotL2 transcription We proceeded to analyse whether AmotL2 positivity overlapped with expression of the hypoxia markers carbonic anhydrase 9 (CA9) or the glucose transporter 1 (refs 25 , 26 ). Immunofluorescent staining of cryosections from colon cancer patients showed a clear overlap between AmotL2 and CAIX, and glucose transporter 1 ( Fig. 2a–c ). We went on to investigate whether AmotL2 was directly transcriptionally controlled by hypoxia. In vitro , 8 h exposure of HeLa cells to 0.3% oxygen (O 2 ) showed AmotL2 positivity in intracellular vesicles in 80% of the cells ( Fig. 3a,b ). The formation of intracellular vesicles was dependent on AmotL2, as treatment with AmotL2 small interfering RNA (siRNA) significantly inhibited hypoxia-induced vesicle formation ( Fig. 3c ). Quantitative Real-Time-PCR (qRT-PCR) analysis of mRNA levels showed that low O 2 levels caused a specific induction of p60 AmotL2 mRNA within 2 h ( Fig. 3d and Supplementary Fig. 2 ). These findings were verified by western blot analysis, showing that HeLa cells under normoxic conditions constitutively express p100, whereas hypoxia preferentially induce the 60 kDa isoform ( Supplementary Fig. 2 ). 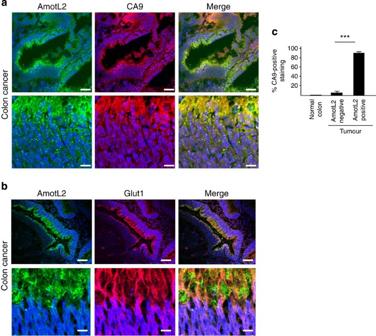Figure 2: AmotL2 expression in hypoxic tumour areas. Immunofluorescent staining of AmotL2 protein expression in colon cancer cryosections show overlap with hypoxic areas in the tumour. (a) AmotL2 expression was detected using antibodies against AmotL2 (green), and low oxygenated tumour areas were visualized using the hypoxia marker carbonic anhydrase 9 (CA9; red). (b) Overlap between AmotL2 (green) and the hypoxia marker glucose transporter 1 (Glut1; red). Scale bars, 200 μm upper panel and 20 μm lower panel. (c) Bar diagram summarizing the percentage of overlap between AmotL2 and CA9 in colon cancer.Pvalues from pairedt-tests, ***P<0.001. Figure 2: AmotL2 expression in hypoxic tumour areas. Immunofluorescent staining of AmotL2 protein expression in colon cancer cryosections show overlap with hypoxic areas in the tumour. ( a ) AmotL2 expression was detected using antibodies against AmotL2 (green), and low oxygenated tumour areas were visualized using the hypoxia marker carbonic anhydrase 9 (CA9; red). ( b ) Overlap between AmotL2 (green) and the hypoxia marker glucose transporter 1 (Glut1; red). Scale bars, 200 μm upper panel and 20 μm lower panel. ( c ) Bar diagram summarizing the percentage of overlap between AmotL2 and CA9 in colon cancer. P values from paired t -tests, *** P <0.001. 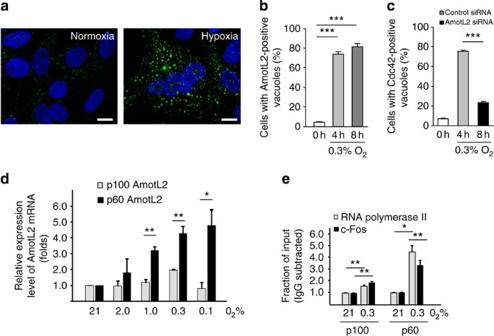Figure 3: Hypoxia activates c-Fos-dependent p60 AmotL2 transcription. (a) Immunofluorescent stainings show induction of AmotL2-positve large vesicles (green) in HeLa cells after 8 h exposure to 0.3% O2. Nuclei were visualized by 4',6-diamidino-2-phenylindole DAPI staining (blue). Scale bars, 10 μm. (b) Bar diagram showing the percentage of cells containing AmotL2-positive vesicles after 4 and 8 h of hypoxia. Data are presented as mean±s.e.m. (n=300). (c) siRNA silencing of AmotL2 inhibits the formation of vesicles. Membranes in vesicles were detected by CDC42 staining and positive vesicles were scored in quadruplicates. Data are presented as mean±s.e.m. (n=300). (d) qPCR analysis ofp60andp100 AmotL2mRNA levels after 8 h exposure to decreasing percentages of O2. (e) Chromatin immunoprecipitation (ChIP) analysis of RNA polymerase II, and c-Fos binding to thep60andp100 AmotL2promoters. Increased binding of both proteins to the p60 promoter was detected after 8 h hypoxia.Pvalues from pairedt-tests; *P<0.05, **P<0.01, ***P<0.001. Each experiment was performed three times. Full size image Figure 3: Hypoxia activates c-Fos-dependent p60 AmotL2 transcription. ( a ) Immunofluorescent stainings show induction of AmotL2-positve large vesicles (green) in HeLa cells after 8 h exposure to 0.3% O 2 . Nuclei were visualized by 4',6-diamidino-2-phenylindole DAPI staining (blue). Scale bars, 10 μm. ( b ) Bar diagram showing the percentage of cells containing AmotL2-positive vesicles after 4 and 8 h of hypoxia. Data are presented as mean±s.e.m. ( n =300). ( c ) siRNA silencing of AmotL2 inhibits the formation of vesicles. Membranes in vesicles were detected by CDC42 staining and positive vesicles were scored in quadruplicates. Data are presented as mean±s.e.m. ( n =300). ( d ) qPCR analysis of p60 and p100 AmotL2 mRNA levels after 8 h exposure to decreasing percentages of O 2 . ( e ) Chromatin immunoprecipitation (ChIP) analysis of RNA polymerase II, and c-Fos binding to the p60 and p100 AmotL2 promoters. Increased binding of both proteins to the p60 promoter was detected after 8 h hypoxia. P values from paired t -tests; * P <0.05, ** P <0.01, *** P <0.001. Each experiment was performed three times. Full size image We then addressed the issue regarding how the p60 AmotL2 gene was transcriptionally controlled. The induction of p60 AmotL2 was independent of hypoxia-inducible factors (HIF)-1α and -2α, as siRNA knockdown of either protein did not affect the upregulation of p60 AmotL2 ( Supplementary Fig. 2 ). To identify potential transcriptional mediators, we searched the ENCODE regulatory data for the AMOTL2 genomic region to identify putative regulatory segments corresponding to the p60 transcript ( http://genome.ucsc.edu/ENCODE/ ). These analyses revealed a single locus located in intron 2 of the p100 transcript that was associated with sequence conservation and also with a DNAse1 hypersensitivity cluster in the human umbilical cord endothelial cell line. We investigated pol II and c-Fos binding at the p100 and p60 promoters in the HeLa and human umbilical cord endothelial cell lines ( Supplementary Fig. 3 ). Binding of c-Fos was observed at the p60 promoter that overlapped with the conserved DNA sequence and the DNase1 hypersensitivity site. c-Fos has been shown to activate target gene transcription in response to various stress signals [27] . Indeed, exposing HeLa cells to 8 h of 0.3% O 2 resulted in a 3.7-fold increase in c-Fos binding as well as 4.6-fold increase in RNA polymerase II indicating activation of transcription ( Fig. 3e ). Taken together, these data indicate that hypoxic regulation of p60 AmotL2 is mediated by c-Fos binding to the p60 AMOTL2 promoter. p60AmotL2 interacts with the TRAPPII complex Immunofluorescent stainings of cDNA-transfected cells showed that whereas p100 AmotL2 localized to cellular junctions, p60 AmotL2 was associated to large vesicles consistent with the staining patterns observed in patient and hypoxic cells in vitro ( Fig. 4a,b ). The origin of these vesicles was not clear as no overlap with endosomal, Golgi, lysosomal or autophagy markers could be detected ( Supplementary Figs 4–7 ). The localization to vesicles was dependent on the C-terminal PDZ-binding motif , as deletion of this site resulted in diffuse cytoplasmic staining ( Fig. 4b ). We used peptides covering the PDZ-binding motif to isolate associated proteins from epithelial cell lysates. Binding proteins were identified by Orbitrap mass spectrometry and the results are listed in Supplementary Table 1 and Supplementary Data 1 and 2 . Interestingly, components of the transport protein particle II complex (TRAPPII) were among the proteins that associated to the AmotL2 PDZ-binding motif ( Fig. 4c ). This complex associated specifically to p60 AmotL2 after 8 h of hypoxia ( Fig. 4d ). Even though the C-terminal PDZ-binding motifs of p100 and p60 AmotL2 are identical, only the latter was associated with TRAPPC9 and 10 ( Fig. 4e ). This may be explained that the N-terminal domain of p100 AmotL2 targets the protein to the cadherin junctional complex (Hultin et al [18] ). Indeed, TRAPPC9 and 10 co-localized with p60 Amotl2 in large vesicles but not with junctional p100 AmotL2 ( Fig. 4f,g ). Overlap of TRAPPC10 with AmotL2-positive vesicles could also be detected in tumours from colon cancer patients ( Fig. 4h ). 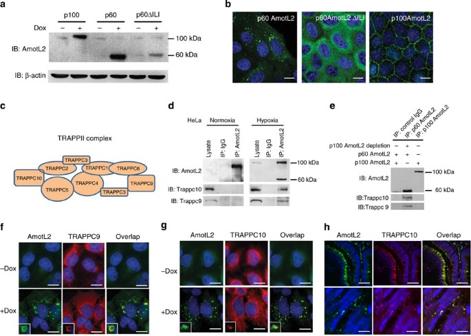Figure 4: The C-terminal PDZ-binding motif of AmotL2 associates to the TRAPPII trans-Golgi membrane transport complex. (a) Western blot analysis showing expression levels of doxycycline (Dox)-regulated p100, p60 and p60 ΔILI (lacking the C-terminal PDZ-binding motif) AmotL2 in MDCK cells. (b) Immunofluorescent stainings showing subcellular localization of transfected p60, p60 ΔILI and p100 AmotL2 (green) in MDCK cells. Scale bars, 10 μm. Note the loss of vacuolar staining in the p60 ΔILI AmotL2 mutant MDCK cells. A peptide corresponding to the last 19 amino acid of AmotL2, and a control peptide containing a 3 amino acid deletion in the C terminus were used for bringing down interacting proteins from HeLa cell lysates. Proteins associated to the peptides were identified by Orbitrap mass spectrometry. The full list of binding proteins is found in theSupplementary Table 1. These data showed that the PDZ-binding motif associates to proteins belonging to the TRAPPII trans-Golgi membrane transport complex. (c) The schematic figure showing the TRAPPII trans-Golgi membrane transport complex. (d) Immunoprecipitation analysis using AmotL2 antibodies. TRAPPC9 and 10 were associated with AmotL2 after 8 h of hypoxia. (e) Co-immunoprecipitation analysis showing specific interaction of TRAPPC9 and 10 with p60AmotL2. (f,g) Immunofluorescence analysis of p60 AmotL2, TRAPPC9 and 10 subcellular localization in Dox-regulated p60AmotL2 HeLa cells. p60AmotL2 co-localizes with TRAPPC9 and 10 in large vesicles (lower panel). Large vesicles showing AmotL2 and Trappc9/Trappc10 double-positive staining are magnified in insets. (h) AmotL2 co-localizes with TRAPPC10 in vesicles in colon cancer specimen. Scale bars, 10 μm. Each experiment was performed three times. Ib, Immunoblot. Figure 4: The C-terminal PDZ-binding motif of AmotL2 associates to the TRAPPII trans-Golgi membrane transport complex. ( a ) Western blot analysis showing expression levels of doxycycline (Dox)-regulated p100, p60 and p60 ΔILI (lacking the C-terminal PDZ-binding motif) AmotL2 in MDCK cells. ( b ) Immunofluorescent stainings showing subcellular localization of transfected p60, p60 ΔILI and p100 AmotL2 (green) in MDCK cells. Scale bars, 10 μm. Note the loss of vacuolar staining in the p60 ΔILI AmotL2 mutant MDCK cells. A peptide corresponding to the last 19 amino acid of AmotL2, and a control peptide containing a 3 amino acid deletion in the C terminus were used for bringing down interacting proteins from HeLa cell lysates. Proteins associated to the peptides were identified by Orbitrap mass spectrometry. The full list of binding proteins is found in the Supplementary Table 1 . These data showed that the PDZ-binding motif associates to proteins belonging to the TRAPPII trans-Golgi membrane transport complex. ( c ) The schematic figure showing the TRAPPII trans-Golgi membrane transport complex. ( d ) Immunoprecipitation analysis using AmotL2 antibodies. TRAPPC9 and 10 were associated with AmotL2 after 8 h of hypoxia. ( e ) Co-immunoprecipitation analysis showing specific interaction of TRAPPC9 and 10 with p60AmotL2. ( f , g ) Immunofluorescence analysis of p60 AmotL2, TRAPPC9 and 10 subcellular localization in Dox-regulated p60AmotL2 HeLa cells. p60AmotL2 co-localizes with TRAPPC9 and 10 in large vesicles (lower panel). Large vesicles showing AmotL2 and Trappc9/Trappc10 double-positive staining are magnified in insets. ( h ) AmotL2 co-localizes with TRAPPC10 in vesicles in colon cancer specimen. Scale bars, 10 μm. Each experiment was performed three times. Ib, Immunoblot. Full size image We and others have shown that the Amot family of proteins interacts with PATJ/Pals1/Lin7 apical polarity protein complex [19] , [28] , [29] . This interaction is mediated by binding to the PDZ-binding motif of AmotL2 as shown in Supplementary Table 1 . The interactions with both p60 and p100 AmotL2 were verified by co-immunoprecipitation analysis. The PATJ/Pals1/Lin7 complex is characteristically associated to the apical membrane protein Crb3. Indeed, transfected cytoplasmic domain Crb3 could be immunoprecipitated in a complex with AmotL2 ( Supplementary Fig. 8 ). Furthermore, immunofluorescence analysis showed a clear overlap between p60 AmotL2 and endogenous Crb3 staining ( Supplementary Fig. 8 ). Par3 was also immunoprecipitated together with AmotL2 and co-localized with p60 AmotL2 in vesicles ( Supplementary Fig. 8 ). Mass spectrometry analysis together with yeast two-hybrid screening revealed that Par3 was directly associated with the PDZ-binding motif of AmotL2 ( Supplementary Table 1 , Supplementary Data 1 and 2 , and Supplementary Fig. 9 ). Furthermore, the use of fluorescence resonance energy transfer (FRET), a method that measures the energy transfer between two chromophores, showed that AmotL2 and Par3 were in close proximity of each other ( Supplementary Fig. 10 ). The activation of doxycycline-regulated p60 AmotL2 resulted in redistribution of Crb3 and Par3 from the apical membrane to intracellular vesicles ( Fig. 5a,b ). This redistribution was not observed with p100 AmotL2. As expected, deletion of the PDZ-binding motif by which Par3 and Crb3 interact with p60 AmotL2 did not affect the subcellular localization of these proteins. ( Fig. 5a,b ). The finding that p60 AmotL2 associates to the TRAPPII complex suggested that this interaction may cause the delocalization of Par3. Indeed, siRNA depletion of the TRAPPII subunit Trappc9 resulted in a similar sequestration of Par3 in intracellular vesicles ( Supplementary Fig. 11 ). 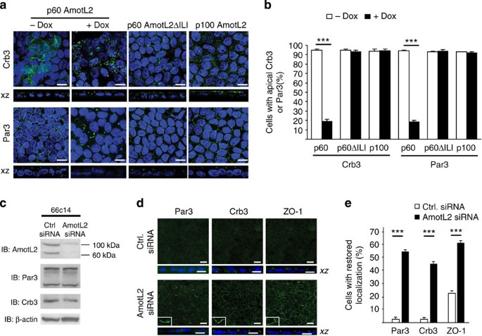Figure 5: p60 AmotL2 sequesters Par3 and Crb3 apical proteins to intracellular large vesicles. (a) The subcellular localization of Crb3 and Par3 in MDCK cells transfected with doxycycline (Dox) inducible p60, p60 ΔILI and p100 AmotL2 was analysed by confocal imaging in thexyandxzaxis as indicated in the figures. (b) Image analysis quantification of apical membrane localization of Crb3 and Par3. Data are presented as mean±s.e.m. (n=500); ***P<0.001 is obtained by pairedt-test. (c) Western blot showing siRNA depletion of AmotL2 in 66c14 cells (mouse breast cancer cell line). (d,e) AmotL2 siRNA knockdown restored polarized localization of Par3, Crb3 and ZO1. Data are presented as mean±s.e.m (n=300). Insets indare high magnification of specific areas in the corresponding low-magnification images. Scale bars, 10 μm.Pvalues from pairedt-tests, ***P<0.001. Each experiment was performed three times. Control, Ctrl. Ib, Immunoblot. Figure 5: p60 AmotL2 sequesters Par3 and Crb3 apical proteins to intracellular large vesicles. ( a ) The subcellular localization of Crb3 and Par3 in MDCK cells transfected with doxycycline (Dox) inducible p60, p60 ΔILI and p100 AmotL2 was analysed by confocal imaging in the xy and xz axis as indicated in the figures. ( b ) Image analysis quantification of apical membrane localization of Crb3 and Par3. Data are presented as mean±s.e.m. ( n =500); *** P <0.001 is obtained by paired t -test. ( c ) Western blot showing siRNA depletion of AmotL2 in 66c14 cells (mouse breast cancer cell line). ( d , e ) AmotL2 siRNA knockdown restored polarized localization of Par3, Crb3 and ZO1. Data are presented as mean±s.e.m ( n =300). Insets in d are high magnification of specific areas in the corresponding low-magnification images. Scale bars, 10 μm. P values from paired t -tests, *** P <0.001. Each experiment was performed three times. Control, Ctrl. Ib, Immunoblot. Full size image We then assessed the cellular consequences of depleting endogenous p60 AmotL2. The metastatic 66c14 tumour cell line is derived from a spontaneous mouse mammary tumour [30] . This cell line expresses endogenous p60 AmotL2 and exhibits a low degree of polarization and cell junction formation. By using siRNA, we depleted p60 AmotL2 expression and analysed the effect on cell polarity ( Fig. 5c ). Downregulation of p60 AmotL2 resulted in re-localization of Par3 and Crb3 to apical junctions and cilia, thus showing that the p60 AmotL2-induced depolarization is reversible. Interestingly, ZO1 could also be detected in cellular junctions after AmotL2 depletion suggesting restoration of tight junctions ( Fig. 5d,e ). Sequestration of Par3 affects tight junction formation Par3 is frequently lost in human cancer, and genetic deletion of Par3 may predispose mice to the formation of breast and skin tumours [14] , [31] , [32] . We therefore investigated whether retention in vesicles would alter the functionality of Par3 molecules. Applying fluorescence recovery after photobleaching, we examined the kinetics of dsred-tagged Par3 localized either to tight junctions or in vesicles. After bleaching a region (~5 μm 2 ), Par3 localized to tight junctions showed rapid recovery of the fluorescent signal ( Fig. 6a,b and Supplementary Fig. 12 ; t 1/2 =11.7±3.2 s, n =12). 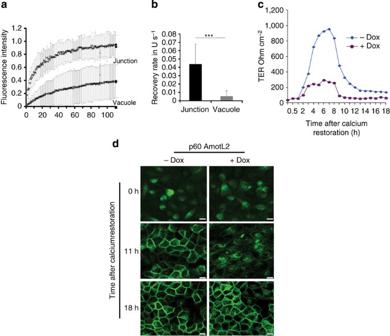Figure 6: p60 AmotL2 affects Par3 dynamics and the kinetics of tight junction formation. (a) Fluorescence recovery after photobleaching analysis of Par3-dsred dynamics in control (Ctrl.) and p60AmotL2-transfected MDCK cells. Par3-dsred fluorescent signals in either cell–cell junctions (control MDCK) or in intracellular large vesicles were bleached and the time to recovery of signal was measured. (b) Bar diagrams shows the recovery rate in U s−1. Par3 junction,n=12; Par3 vacuole,n=11. Error bars represent s.d.. Student’st-test and thePvalues were <0.000072 for the two-tailed test. (c) Analysis of the kinetics of junction formation in MDCK cells transfected with doxycycline (Dox)-regulated p60AmotL2. MDCK cells were calcium depleted and the kinetics of trans-epithelial resistance (TER) after re-addition of calcium was markedly affected by Dox-induced p60 AmotL2 expression in MDCK cells. (d) Immunofluorescent stainings of E-cadherin 0, 11 and 18 h after re-addition of calcium. The targeting of E-cadherin to cell–cell junctions is severely delayed in Dox-induced p60AmotL2 MDCK cells. Scale bars, 10 μm. Each experiment was performed three times. Figure 6: p60 AmotL2 affects Par3 dynamics and the kinetics of tight junction formation. ( a ) Fluorescence recovery after photobleaching analysis of Par3-dsred dynamics in control (Ctrl.) and p60AmotL2-transfected MDCK cells. Par3-dsred fluorescent signals in either cell–cell junctions (control MDCK) or in intracellular large vesicles were bleached and the time to recovery of signal was measured. ( b ) Bar diagrams shows the recovery rate in U s −1 . Par3 junction, n =12; Par3 vacuole, n =11. Error bars represent s.d.. Student’s t -test and the P values were <0.000072 for the two-tailed test. ( c ) Analysis of the kinetics of junction formation in MDCK cells transfected with doxycycline (Dox)-regulated p60AmotL2. MDCK cells were calcium depleted and the kinetics of trans-epithelial resistance (TER) after re-addition of calcium was markedly affected by Dox-induced p60 AmotL2 expression in MDCK cells. ( d ) Immunofluorescent stainings of E-cadherin 0, 11 and 18 h after re-addition of calcium. The targeting of E-cadherin to cell–cell junctions is severely delayed in Dox-induced p60AmotL2 MDCK cells. Scale bars, 10 μm. Each experiment was performed three times. Full size image Previous reports have shown that silencing of Par3 alters the kinetics of tight junction formation [33] . The integrity of tight junctions in an epithelial layer can be analysed by measuring the trans-epithelial resistance. The kinetics of the reformation of cellular junctions can be monitored after re-addition of calcium in calcium-depleted cells. Similar to what was observed with loss of Par3, sequestration of Par3 in vesicles resulted in a significantly delayed formation of tight junctions as well as delayed transport of E-cadherin to cell junctions ( Fig. 6c,d and Supplementary Fig. 12 ). p60 AmotL2 disrupts apical–basal polarity Our findings raised the question whether the ectopic localization of Par3 and Crb3 to vesicles also would result in a general loss of targeting of proteins to either the apical or basal compartments. To address this issue, epithelial cells were grown on Matrigel-coated trans-well filters polarize with clearly distinguishable apical and basal membrane compartments [34] . The distribution of proteins was analysed by immunofluorescent staining for ezrin (apical membrane marker), E-cadherin (lateral membrane marker) and β-catenin (baso-lateral marker). Expression of p60 AmotL2 clearly caused scrambling of these membrane markers, which now could be detected in basal, lateral and apical–basal membranes ( Fig. 7a,b and Supplementary Fig. 12 ). The hepatocyte growth factor (HGF) signalling via its receptor, c-Met, is closely associated to tumour invasion and metastasis [35] . Interestingly, p60 AmotL2 expression resulted in delocalization of c-Met from junctions to apical and basal membrane compartments ( Fig. 7a,b ). We further analysed the correlation between AmotL2 expression and loss of polarity in colon cancer. Polarity was assessed using the Golgi marker gm130 that visualizes the Golgi apparatus that is localized on the apical side between the epithelial nuclei and the apical lumen in polarized epithelia ( Fig. 7c ). Double staining showed a positive correlation between loss of polarity and AmotL2 expression ( Fig. 7d ). 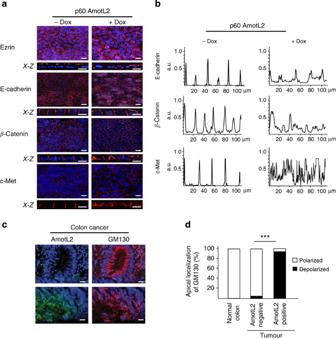Figure 7: p60 AmotL2 disrupts apical–basal sorting of membrane proteins. (a) MDCK cells transfected with doxycycline (Dox)-regulated p60 AmotL2 were grown on trans-well filters for 5 days. Filters were stained using antibodies against Ezrin (apical membrane), E-cadherin (lateral membrane), β-catenin (baso-lateral membrane) and c-Met (lateral membrane). Images in thexzaxis showed loss of defined apical and basal domains in p60 AmotL2-induced cells. Scale bars,10 μm. (b) Linear diagrams showing the delocalization of E-cadherin, β-catenin and c-Met from cellular junctions to a more uniform membrane location after p60 AmotL2 induction. (c) AmotL2 expression is associated with loss of polarity in colon cancer. A GM130 antibody detecting the Golgi apparatus was used to assess polarity in AmotL2-negative (top panel) and AmotL2-positive tumour areas (bottom panel). Scale bars, 10 μm. (d) The percentage of tumour cells with maintained apical–basal polarity was negatively correlated with AmotL2 expression. Data are presented as mean±s.e.m. (n=600); ***P<0.001 is obtained by pairedt-test. Size bars, 10 μm. Each experiment was performed three times. Figure 7: p60 AmotL2 disrupts apical–basal sorting of membrane proteins. ( a ) MDCK cells transfected with doxycycline (Dox)-regulated p60 AmotL2 were grown on trans-well filters for 5 days. Filters were stained using antibodies against Ezrin (apical membrane), E-cadherin (lateral membrane), β-catenin (baso-lateral membrane) and c-Met (lateral membrane). Images in the xz axis showed loss of defined apical and basal domains in p60 AmotL2-induced cells. Scale bars,10 μm. ( b ) Linear diagrams showing the delocalization of E-cadherin, β-catenin and c-Met from cellular junctions to a more uniform membrane location after p60 AmotL2 induction. ( c ) AmotL2 expression is associated with loss of polarity in colon cancer. A GM130 antibody detecting the Golgi apparatus was used to assess polarity in AmotL2-negative (top panel) and AmotL2-positive tumour areas (bottom panel). Scale bars, 10 μm. ( d ) The percentage of tumour cells with maintained apical–basal polarity was negatively correlated with AmotL2 expression. Data are presented as mean±s.e.m. ( n =600); *** P <0.001 is obtained by paired t -test. Size bars, 10 μm. Each experiment was performed three times. Full size image Amot was first described as the founding member of the Amot family [36] . Similar to AmotL2, Amot consists of two isoforms where the shorter version contains a coiled-coil domain and a C-terminal PDZ-binding motif ( Supplementary Fig. 13 ). Expression of the p80Amot isoform in MDCK cells did not, however, negatively affect apical–basal polarity ( Supplementary Fig. 13 ). This argues that the anti-polarity effects are inherent to p60 AmotL2. MDCK as well as Caco-2 cells form polarized cysts when grown in 3D matrices consisting of Matrigel or collagen. Single cells immersed in Matrigel formed polarized cysts within 4 days of culture ( Fig. 8a ). Doxycycline-mediated induction of p60 AmotL2, but not p100 AmotL2 or p60 AmotL2 ΔILI mutant, inhibited lumen formation and resulted in loss of apical–basal polarity ( Fig. 8b,c ). This effect was reversible as removal of doxycycline restored the ability to polarize and form an apical lumen ( Fig. 8d ). These data show that activation of p60 AmotL2 interferes with proper sorting of membrane proteins that results in a reversible loss of cellular architecture in vitro . 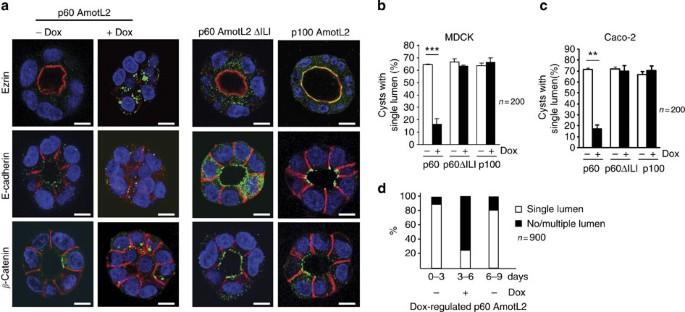Figure 8: p60 AmotL2 inhibits cyst formationin vitro. (a) As shown in the control (doxycycline, −Dox.), MDCK cells polarize and form an apical lumen after 4 days of 3D culture in Matrigel, extracellular matrix derived from the Engelbreth–Holm–Swarm tumour cells. Cysts were stained for AmotL2 (green) and the apical membrane protein ezrin (red), lateral membrane marker E-cadherin (red) and the baso-lateral membrane β-catenin (red). Induction of p60 AmotL2 resulted in re-localization of the observed markers to lateral, basal and apical membrane compartments. Scale bars, 10 μm. (b,c) Inhibition of lumen formation in MDCK and Caco-2 cysts grown in Matrigel is summarized in a bar diagram. Data are mean±s.e.m. (n=200),Pvalues from pairedt-tests; **P<0.01, ***P<0.001. (d) Reversible inhibition of cyst formation by p60 AmotL2. The bar diagram shows the frequency of single lumen formation of MDCK cells after 3 days in Matrigel (3 days). Activation of p60 AmotL2 expression efficiently inhibited lumen formation (6 days). Removal of Dox restored the capacity to form cysts with single lumens (9 days). Data are mean±s.e.m. (n=900). ***P<0.001 is obtained by pairedt-test. Each experiment was performed three times. Figure 8: p60 AmotL2 inhibits cyst formation in vitro. ( a ) As shown in the control (doxycycline, −Dox. ), MDCK cells polarize and form an apical lumen after 4 days of 3D culture in Matrigel, extracellular matrix derived from the Engelbreth–Holm–Swarm tumour cells. Cysts were stained for AmotL2 (green) and the apical membrane protein ezrin (red), lateral membrane marker E-cadherin (red) and the baso-lateral membrane β-catenin (red). Induction of p60 AmotL2 resulted in re-localization of the observed markers to lateral, basal and apical membrane compartments. Scale bars, 10 μm. ( b , c ) Inhibition of lumen formation in MDCK and Caco-2 cysts grown in Matrigel is summarized in a bar diagram. Data are mean±s.e.m. ( n =200), P values from paired t -tests; ** P <0.01, *** P <0.001. ( d ) Reversible inhibition of cyst formation by p60 AmotL2. The bar diagram shows the frequency of single lumen formation of MDCK cells after 3 days in Matrigel (3 days). Activation of p60 AmotL2 expression efficiently inhibited lumen formation (6 days). Removal of Dox restored the capacity to form cysts with single lumens (9 days). Data are mean±s.e.m. ( n =900). *** P <0.001 is obtained by paired t -test. Each experiment was performed three times. Full size image p60 AmotL2 potentiates the response to HGF Loss of polarity has been tightly coupled to the acquisition of an invasive phenotype [12] , [14] . To test whether activation of p60 AmotL2 would promote invasion, Caco-2 and MDCK cells transfected with doxycycline-regulated p60 AmotL2 were embedded in Matrigel. Analysis of cellular invasion by phalloidin staining showed that p60 AmotL2-induced depolarization was not sufficient to induce an invasive phenotype in these settings ( Fig. 9a and Supplementary Fig. 14 ). As previously shown in Fig. 7a , p60 AmotL2 induced a marked change in the membrane localization of c-Met. This finding raised the question whether re-localization of c-Met potentiated the response to HGF. This was indeed the case as the addition of HGF to p60 AmotL2-depolarized cells induced a robust invasive response in both MDCK and Caco-2 cysts ( Fig. 9a,b and Supplementary Fig. 14 ). The potentiation of the invasive response appeared to be independent of epithelial–mesenchymal transition as markers of the process remained unaffected ( Supplementary Fig. 15 ). As previously reported, the 66c14 tumour cells are highly invasive in vitro and in vivo [37] . When embedded in Matrigel, 90% of the cells form spheroids with massive invasion into the surrounding matrix ( Fig. 9c,d ). The invasive properties could be abrogated by depleting AmotL2 expression using short hairpin RNA ( Fig. 9c,d ). Stimulation of the 66c14 cells with HGF increased invasion of the control cells, whereas AmotL2-depleted cells remained unresponsive ( Fig. 9c,d ). Taken together, these data show that depolarization and consequently re-localization of c-Met increases the invasive response to HGF stimulation. 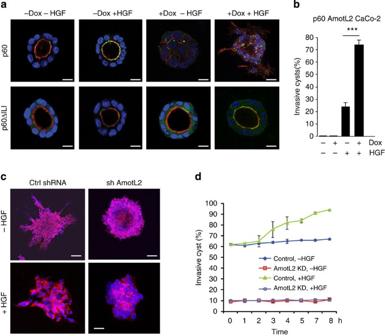Figure 9: p60 AmotL2 potentiates the invasive response to hepatocyte growth factor (HGF)in vitro. (a) Caco-2 cells transfected with doxycycline (Dox)-regulated p60 or p60 ΔILI AmotL2 were grown in Matrigel in the presence or absence of HGF (5 ng ml−1) as indicated. Cysts were analysed with immunofluorescent staining using AmotL2 antibodies (green), actin was visualized by phalloidin staining (red) and nuclei are stained with 4',6-diamidino-2-phenylindole (blue). HGF promoted invasion in depolarized p60 AmotL2 expressing cysts. Scale bars, 10 μm. (b) Bar diagram shows the percentage of invasive Caco-2 cysts grown in the presence or absence of Dox and HGF as indicated. Data are presented as mean±s.e.m. (n=200); ***P<0.001 is obtained by pairedt-test. (c) shRNA depletion of AmotL2 in 66cl4 cells reverted their invasive phenotype and their ability to respond to HGF stimulation. 66cl4 cells were cultured in 3D Matrigel for 3 days and visualized by phalloidin actin staining (red). Scale bars, 10 μm. (d) AmotL2-depleted cells remained unresponsive to HGF stimulation. Data are mean±s.e.m. (n=300). Control, Ctrl. Figure 9: p60 AmotL2 potentiates the invasive response to hepatocyte growth factor (HGF) in vitro . ( a ) Caco-2 cells transfected with doxycycline (Dox)-regulated p60 or p60 ΔILI AmotL2 were grown in Matrigel in the presence or absence of HGF (5 ng ml −1 ) as indicated. Cysts were analysed with immunofluorescent staining using AmotL2 antibodies (green), actin was visualized by phalloidin staining (red) and nuclei are stained with 4',6-diamidino-2-phenylindole (blue). HGF promoted invasion in depolarized p60 AmotL2 expressing cysts. Scale bars, 10 μm. ( b ) Bar diagram shows the percentage of invasive Caco-2 cysts grown in the presence or absence of Dox and HGF as indicated. Data are presented as mean±s.e.m. ( n =200); *** P <0.001 is obtained by paired t -test. ( c ) shRNA depletion of AmotL2 in 66cl4 cells reverted their invasive phenotype and their ability to respond to HGF stimulation. 66cl4 cells were cultured in 3D Matrigel for 3 days and visualized by phalloidin actin staining (red). Scale bars, 10 μm. ( d ) AmotL2-depleted cells remained unresponsive to HGF stimulation. Data are mean±s.e.m. ( n =300). Control, Ctrl. Full size image p60 AmotL2 promotes tumour formation and invasion in vivo We further assessed the role of p60 AmotL2 on tumour invasion in mice. Control or p60 AmotL2 expressing Caco-2 cells were co-injected with NIH3T3 cells in order to promote tumour take. Histological analysis showed that control tumours grew as polarized glandular epithelia ( Fig. 10a,c ), whereas these structures were completely lost in p60 AmotL2 expressing tumours ( Fig. 10b,d,f ). Both control and p60 AmotL2-transfected tumours grew at a similar rate ( Fig. 10e ). The p60 AmotL2 tumours exhibited massive infiltration in surrounding adipose tissue ( Fig. 10d,g ). Increase of tumour DNA was also present in blood from animals with p60 AmotL2 expressing tumours ( Fig. 10h ). We also assessed whether silencing of endogenous AmotL2 affected tumour growth and dissemination in vivo . 66c14/control or 66c14/shAmotL2 cells were injected orthotopically in the mammary fat pad of Balb/c mice, and tumour progression was followed by luciferase imaging. As shown in Fig. 10i,j , control tumours grew rapidly and all animals were euthanized within 50 days after injection after reaching a tumour size of 10 mm in diameter. In contrast, 66c14/shAmotL2 cells were detectable by luciferase imaging but did not grow to a palpable size. Taken together, our results show that p60 AmotL2 controls tissue architecture, response to invasive cues and consequently tissue invasion and tumour growth. 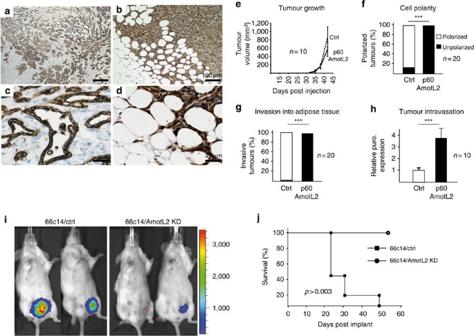Figure 10: p60 AmotL2 promotes tumour growth and invasionin vivo. (a–d) Caco-2 tumours were co-injected with NIH3T3 fibroblasts subcutaneously in SCID mice. Tumours were resected, embedded in paraffin and analysed by histochemical staining using pan-Keratin antibodies. (a,c) Panels show the villous, polarized growth pattern of control (Ctrl) Caco-2 tumours. Note the distinct apical lumen formation inc. (b) Tumours from p60 AmotL2 expressing Caco-2 cells completely lacked polarized structures and invaded into surrounding adipose tissues as shown in high magnification ind. (e) Graphs show tumour growth days after injection. No significant difference in growth rate could be detected. (f) Bar diagram shows the percentage of tumours with polarized villous structures. Data are presented as mean±s.e.m. (n=20); ***P<0.001 is obtained by pairedt-test. (g) Bar diagram shows the percentage of tumours containing cytokeratin-positive cells in the adipose tissue adjacent to the primary tumour. Data are presented as mean±s.e.m. (n=20); ***P<0.001 is obtained by pairedt-test. (h) Quantification of tumour DNA in blood. Relative levels of tumour DNA was detected by qPCR with primers targeting plasmid DNA. Data are presented as mean±s.e.m. (n=10); ***P<0.001 is obtained by pairedt-test. (i) Representative IVIS images of mice, 29 days (Ctrl shRNA) or 49 days (Amotl2 shRNA KD) after injection of 66C14 cells in the mammary fat pad. The relationship between colour and light intensity in arbitrary units (counts) for the whole animal images is given by the colour bar at the right side of the figure. (j) Kaplan–Meier survival curve for tumour-free survival of mice injected with Ctrl shRNA (n=7) or Amotl2 shRNA KD (n=6).Pvalue was calculated with a log-rank test. Each experiment was performed three times. Puromycin, Puro. Figure 10: p60 AmotL2 promotes tumour growth and invasion in vivo. ( a – d ) Caco-2 tumours were co-injected with NIH3T3 fibroblasts subcutaneously in SCID mice. Tumours were resected, embedded in paraffin and analysed by histochemical staining using pan-Keratin antibodies. ( a , c ) Panels show the villous, polarized growth pattern of control (Ctrl) Caco-2 tumours. Note the distinct apical lumen formation in c . ( b ) Tumours from p60 AmotL2 expressing Caco-2 cells completely lacked polarized structures and invaded into surrounding adipose tissues as shown in high magnification in d . ( e ) Graphs show tumour growth days after injection. No significant difference in growth rate could be detected. ( f ) Bar diagram shows the percentage of tumours with polarized villous structures. Data are presented as mean±s.e.m. ( n =20); *** P <0.001 is obtained by paired t -test. ( g ) Bar diagram shows the percentage of tumours containing cytokeratin-positive cells in the adipose tissue adjacent to the primary tumour. Data are presented as mean±s.e.m. ( n =20); *** P <0.001 is obtained by paired t -test. ( h ) Quantification of tumour DNA in blood. Relative levels of tumour DNA was detected by qPCR with primers targeting plasmid DNA. Data are presented as mean±s.e.m. ( n =10); *** P <0.001 is obtained by paired t -test. ( i ) Representative IVIS images of mice, 29 days (Ctrl shRNA) or 49 days (Amotl2 shRNA KD) after injection of 66C14 cells in the mammary fat pad. The relationship between colour and light intensity in arbitrary units (counts) for the whole animal images is given by the colour bar at the right side of the figure. ( j ) Kaplan–Meier survival curve for tumour-free survival of mice injected with Ctrl shRNA ( n =7) or Amotl2 shRNA KD ( n =6). P value was calculated with a log-rank test. Each experiment was performed three times. Puromycin, Puro. Full size image Hypoxia is an important component of the tumour microenvironment that promotes tumour expansion by stimulating growth of stromal cells and blood vessel formation. Hypoxia also affects the gene expression pattern of the tumour cells directly causing increased heterogeneity and a selection of invasive metastatic cells [38] . Previous findings have shown that hypoxia triggers a de-differentiated stem cell-like phenotype in neuroblastoma cells as well as upregulates the tyrosine kinase receptors such as c-Met, thereby making the cells susceptible to invasive cues [35] , [39] . By the application of chromatin immunoprecipitation (ChIP) analysis, we identified p60 AmotL2 as a novel target gene for c-Fos-mediated transcription. c-Fos is part of the AP1 transcriptional complex that is induced by variety of stimuli such as growth factors, hormones as well as infections, and physical or chemical stress. c-Fos has also been shown to be activated by ischaemia in the heart and brain [27] , [40] . The AP1 complex has mainly been shown to be involved in proliferation, cell death and cellular transformation. However, a role in the control of cell polarity has also been proposed. This was based on findings that activation of c-Fos or its partner c-Jun negatively regulated apical–basal polarity in MDCK cells [41] , [42] . We show in this paper that p60 AmotL2 is a transcriptional target gene of c-Fos, and thus provide a plausible mechanism how c-Fos negatively regulates cell polarity. The continuous maintenance of cell apical and basal membranes, as well as cell junctions is highly dynamic and dependent on vesicular transport, and the internalization and recycling of proteins. Interference with the sorting and recycling of proteins may thus perturb cellular polarity [43] . In this report, we show that p60 AmotL2 interferes with apical transport of the Par3 and Crb3 proteins. We provide evidence that this is mediated through the interaction with the TRAPPII trans-Golgi complex. The TRAPPII is a highly conserved tethering complex that binds to Golgi-derived (coat protein complex 1-coated) vesicles to mediate Golgi traffic and has been implicated in the selective transport of proteins to the plasma membrane in polarized cells [44] , [45] . The p60 AmotL2 vesicles are stationary within the cytoplasm as opposed to p100 AmotL2 vesicles. Our data suggest a model in which p60 AmotL2 inactivates TRAPPII, and thereby inhibit apical transport of polarity proteins, which then disrupts cell polarity. Whether p60 AmotL2 affects the guanine nucleotide exchange factor activity of the TRAPPII complex remains to be shown. However, little is known whether the deregulation of polarity proteins is caused by inactivation by functional mutations or downregulation of expression. Our findings point to a third possibility where local stress signals are interpreted by epithelial cells that are then responding by p60 AmotL2 expression. The intracellular sequestration of the polarity proteins may be reversed when p60 AmotL2 expression is lost, thus indicating a high degree of plasticity in the maintenance of the polarized state. We also show that disruption of polarity does not in itself trigger invasive properties but potentiates the pro-migratory/invasive response to HGF. Our data show that the HGF receptor, c-Met, co-localizes with E-cadherin in polarized cells, which is consistent with previous findings. However, p60 AmotL2 expression disrupts the c-Met localization to the membrane micro-domain, and thus allow c-Met molecules to translocate to apical and basal membranes. Whether this makes the receptor more accessible for binding to the HGF ligand or whether the receptor is more prone to activation outside the lateral membrane domains remains to be shown. Our data are consistent with recent studies where loss of Lgl2 cooperated with HER2 activation to induce an invasive phenotype in zebrafish and mammary epithelia [46] . Recent publications have implicated the Amot family of proteins as regulators of the HIPPO pathway. Amot, AmotL1 and AmotL2 all contain WW-binding motifs that interact with the Yap1 oncoprotein, which is then retained in the cellular junctions [47] , [48] , [49] . This suggests a tumour-suppressive role of p100 AmotL2. Our data support an independent role of the p60 isoform in promoting tumour progression since the p60 isoform lacks the WW-binding motif and thus does not retain Yap1 in the cytoplasm ( Supplementary Fig. 15 ). The invasive front of metastatic tumours typically contains cells that escaped from their original context and lost apical–basal polarity. We present a direct molecular mechanism how these cells respond to local stress signals that cause mislocalization of the Par3 and Crb3 polarity complexes. This provides another perspective on how cells gain a plastic phenotype that is not mutually exclusive to that of epithelial–mesenchymal transition. This should add insight on how cells are driven towards a metastatic pathway, which hopefully could be interfered with in the future. Patient samples The patient studies were approved by the Karolinska Hospital, Research Ethics Committee, (2012/90-31/2, 00-229 and 2010/0066-32), and informed consent was obtained from all participants. Patients included in the breast study were diagnosed with stages I–III breast cancers and were operated according to the sentinel-node technique (tumour and draining lymph node were resected in parallel) at Karolinska University Hospital during 2001–2003. No patient received neo-adjuvant therapy. All primary tumours and lymph nodes were histopathologically evaluated independently by two board certified clinical pathologists. Patients in the colon study were operated during 1993–1996 at the Ersta Hospital, Stockholm. The study was limited to patients classified as Dukes A–C. All cases selected were original histopathological diagnosis, and the original haematoxylin and eosin-stained sections were re-examined by two board certified clinical pathologists. Animal studies Animal experiments were performed according to a permit from the Stockholm South ethical committee in Sweden. SCID and Balb/C mice of 6- to 8-week old were used for tumour injection. Tumour development was monitored and tumour size was measured every other day with calipers. The mice were monitored biweekly for tumour development and fluorescence was measured by IVIS Xenogen Spectrum after intraperitoneal luciferin-D injection (150 mg kg −1 ). Cell culture HeLa, MDCK, Caco-2 and NIH3T3 cells (American Type Culture Collection) were cultured in dulbecco's modified eagle medium (DMEM) medium (Sigma) supplemented with 10% fetal calf serum (Gibco), 1% glutamine and 1% penicillin/streptomycin (Gibco). MDCK and Caco-2 cells were plated on trans-well polycarbonate filters of 0.4 μm pore size (Corning Costar) at a density of 2.5 × 10 5 cells cm −2 in order to establish apical–basal polarity. Immunohistochemical staining The tumour section slides were deparaffinized in xylene and rehydrated in ethanol. Thereafter, the slides were incubated in 3% hydrogen peroxide to inhibit the endogenous peroxidase activity. Antigen retrieval was carried out in citrate buffer (pH 6.0) for 20 min in a microwave oven followed by 20 min of cooling at room temperature. In order to reduce nonspecific background staining, the slides were blocked with horse serum followed by an overnight incubation at 4 °C with the AmotL2 polyclonal antibody (1:400) antibody. The samples were then rinsed and incubated with biotinylated horse anti-mouse secondary antibodies, and thereafter rinsed and incubated with avidin–biotin–peroxidase complexes. Visualization of immunostaining was achieved by immersion in 0.05% 3,3′-diaminobenzidine tetrahydrochloride followed by counterstaining with haematoxylin. Tissues were scored, and were examined blinded to clinical and pathological data (L.H.). Immunohistochemical staining intensity was defined by a visual grading scale 0–2 based on intensity as well as focal extent (grade 0=no staining, grade 1<25 positivity and grade 2>25%). Survival rates were estimated by applying Kaplan–Meier statistics and rated for their significance calculating the log-rank test. Cross-tabulations were calculated using the χ 2 -test. Hypoxia exposure Cells grown in Petri dishes or chamber slides were exposed to 2, 1, 0.3 or 0.1% O 2 for 0–16 h in a hypoxia chamber (Galaxy 48 R, New Brunswick). The medium used during the hypoxia treatment was degassed with a gas mixture consisting of 95% nitrogen and 5% carbon dioxide (AGA AB, Sweden), and was added to cells before start of hypoxic exposure. Quantitative real-time PCR Real-time PCR was performed to quantify AmotL2 expression in hypoxia-exposed HeLa cells as well as puromycin expression (marker for the stable transfected Caco-2 tumour cells) from the blood of tumour bearing mice. Total RNA was extracted by RNeasy mini kit (Qiagen) according to the manufacturer’s instructions. Purified RNA was treated with RNase-free DNaseI to ensure complete degradation of potential genomic DNA contamination, followed by the addition of 25 mM EDTA and heat denaturation of the enzyme. RNA samples were reverse transcribed to cDNA with random hexamer primers using a SuperScript III First-Strand cDNA Synthesis Kit (Invitrogen). Real-time PCR primers were designed with RealTimeDesign software ( http://www.biosearchtech.com ) and were custom made by ThermoScientific. The real-time PCR was carried out on an ABI PRISM 7900 System (Applied Biosystems) according to the manufacturer’s instructions with a 25-μl reaction volume containing 25 ng of cDNA templates. The sequence of the primers used in real-time PCR is human AmotL2, 5′-CACAGGCATCAGGAGATGGAAAG-3′ (forward), and 5′-GCGCTGCTGAAGGACCTTG-3′ (reverse); human p60 AmotL2, 5′-CTCTGCTGTCTGACTCTTGC-3′ (forward), and 5′-GCAGATTCCAATCTCTCTC-3′ (reverse); human p100 AmotL2, 5′-TTGTGGTTCGCTTTGATCCC-3′ (forward), and 5′-CGCAGTCAGACACCACAACC-3′ (reverse); puromycin, 5′-ACAGATGGAAGGCCTCCTG-3′ (forward), and 5′-CAGACCCTTGCCCTGGTG-3′ (reverse); human β-actin, 5′-GCGGGAAATCGTGCGTGACATT-3′ (forward) and 5′-GATGGAGTTGAAGGTAGTTTCGTG-3′ (reverse). Mouse β-actin primer was purchased from Qiagen (cat. no. QT01136772). Each sample was run in triplicate. The amplification of β-actin was used as a control to normalize the expression level of AmotL2 and puromycin between samples. Negative controls without template were always included as negative controls. Dissociation analysis was performed at the end of each run to confirm the specificity of the reaction. The real-time qPCR results were analysed with a ΔΔ C t method. Western blotting Proteins separated by SDS-PAGE were transferred to nitrocellulose membrane (Waterman). Nonspecific antibody binding was blocked with 5% milk in PBS buffer containing 0.1% Tween 20 and membranes were incubated with primary antibody for 2 h at room temperature. Species-specific horseradish peroxidase-conjugated secondary antibodies were used for detection of the primary antibodies and were developed with a chemiluminescent substrate according to the manufacturer’s instructions (PerkinElmer). Full blots are shown in Supplementary Figs 16 and 17 . Chromatin immunoprecipitation ChIP was carried out using the ChIP assay Kit (Upstate/Millipore, cat. no. 17–295) according to the manufacturer’s recommendations. In brief, 80–90% confluent HeLa cells were exposed to 0.3% O 2 in a hypoxic incubator for 8 h followed by crosslinking in 1% formaldehyde. The lysates were sonicated with a Bioruptor Sonicator (Diagenode): 30 s ON/30 s OFF, setting=high, 18 cycles. The sonicated samples were pre-cleared with Salmon Sperm DNA/Protein A Agarose (Life Technologies, Carlsbad, CA, USA, cat. no. 16-157C). A quantity of 4 μg of antibody was used per sample and incubated for 16 h on a rotating platform at 4 °C. The DNA was eluted in a two-step procedure using 150 μl of freshly prepared ‘elution buffer’ (1% SDS and 100 mM NaHCO 3 ) and the crosslinking was reversed. The DNA was finally eluted using Qiagen PCR purification kit (Qiagen, cat. no. 28106) according to the manufacturer’s recommendations. The eluted DNA was analysed on qRT-PCR using the KAPA 2G SyberGreen (Kapa Biosystems, Woburn, MA, USA, cat. no. KK4605) on the Applied Biosystem 7900HT platform with the following conditions: 95 °C, 3 min; 95 °C, 3 s; and 60 °C 30 s. The primer sets targeting AmotL2 p100 and p60 promoters are: 5′-GGGAACCTGAAACTCTCACATTCC-3′ (AmotL2 p100 promoter forward); 5′-GGCGGCGAAGATGTGTTCTC-3′ (AmotL2 p100 promoter reversed); 5′-GTGAAGGGAAAGGAGTTGCTATTC-3′ (AmotL2 p60 promoter forward); 5′-CAGGCAGACACAACTGGCATTC-3′ (AmotL2 p60 promoter reversed). The antibodies used for the ChIPs were polymerase II (Santa Cruz, Santa Cruz, CA, USA, cat. no. sc899x) and c-Fos (Santa Cruz, Santa Cruz, CA, USA, cat. no. sc-52x). Peptide pull-down Peptides corresponding to full-carboxyl terminal sequence of mouse AmotL2 DSIAATRVQDLSDMVEILI or lacking the last three amino acids involved in PDZ-binding domain were synthesized (Innovagen, Lund, Sweden) and crosslinked to N-hydroxysuccinimide-activated Sepharose 4 Fast Flow beads according to the manufacturer’s instructions (GE Healthcare). Pull-down experiments were performed using Caco-2 and Hela cell lysates. In brief, cells were grown until 90% confluence and lysed in 50 mM HEPES, pH 7.5, 1 mM EGTA, 150 mM NaCl, 1.5 mM MgCl 2 , 10% glycerol and 1% Triton X-100 containing phosphates and proteases inhibitors. Beads containing full-length or truncated peptides (20 μl) or control beads prepared without peptides were added to soluble cell lysates (1 ml, 5 mg ml −1 ) and incubated for 2 h at 4 °C. Beads were washed in lysis buffer (50 mM HEPES, pH 7.5, 1 mM EGTA, 150 mM NaCl, 1.5 mM MgCl 2 , 10% glycerol and 1% Triton X-100). For quality control, 10% of proteins bound to beads were loaded, separated on NuPAGE 4–12% Bis-tris acrylamide gels in Mops buffer according to the manufacturer’s instructions (Invitrogen and Life Technologies), and protein complexes were visualized after silver staining. For mass spectrometry analysis, pull-down proteins extracts (90%) were loaded on NuPAGE 4–12% Bis-tris acrylamide gels. Running of samples was stopped as soon as proteins were stacked as a single band. Protein containing bands were stained with Thermo Scientific Imperial Blue, cut from the gel, and following reduction and iodoacetamide alkylation, and digested with high-sequencing grade trypsin (Promega, Madison, WI, USA). Extracted peptides were concentrated before mass spectrometry analysis. Mass spectrometry Mass spectrometry analysis were carried out by Liquid chromatography-tandem Mass Spectrometry using a LTQ-Velos-Orbitrap (Thermo Electron, Bremen, Germany) connected to a nanoLC Ultimate 3000 Rapid Separation Liquid chromatography system (Dionex, Sunnyvale, CA, USA). Five microlitres corresponding to 20% of whole sample were injected on the system. After pre-concentration and washing of the sample on a Dionex Acclaim PepMap 100 column (C18, 2 cm × 100 μm i.d., 100 A pore size, 5 μm particle size), peptides were separated on a Dionex Acclaim PepMap RSLC column (C18, 15 cm × 75 μm i.d., 100 A pore size, 2 μm particle size) at a flow rate of 300 nl min −1 with a two-step linear gradient (4–20% acetonitrile/H 2 O, 0.1% formic acid for 90 min; and 20–45% acetonitrile/H 2 O, 0.1% formic acid for 30 min). The separation of the peptides was monitored by a UV detector (absorption at 214 nm). For peptides ionization in the nanospray source, spray voltage was set at 1.4 kV and the capillary temperature at 275 °C. All samples were measured in a data-dependent acquisition mode. Each run was preceded by a blank MS run in order to monitor system background. The peptide masses were measured in a survey full scan (scan range 300–1700 m/z , with 30 K full width at half maximum resolution at m/z =400, target automatic gain control value of 1.00 × 106 and maximum injection time of 500 ms). In parallel to the high-resolution full scan in the Orbitrap, the data-dependent CID scans of the 10 most intense precursor ions were fragmented and measured in the linear ion trap (normalized collision energy of 35%, activation time of 10 ms, target AGC value of 1.00 × 104, maximum injection time 100 ms and isolation window 2 Da). Parent masses obtained in orbitrap analyser were automatically calibrated on the 445.120025 ion used as lock mass. The fragment ion masses were measured in the linear ion trap to have a maximum sensitivity and the maximum amount of MS/MS data. Dynamic exclusion was implemented with a repeat count of 1 and exclusion duration of 30 s. Data analysis : Raw files generated from mass spectrometry analysis were processed with Proteome Discoverer 3.1 (Thermo Fisher Scientific). This software was used to search data via in-house Mascot server (version 2.4.1; Matrix Science Inc., London, UK) against the Human database subset (20,271 sequences) of the SwissProt database (version 2014-02). For the database search, the following settings were used: a maximum of one miscleavage, oxidation as a variable modification of methionine, carbamido-methylation as a fixed modification of cysteine and trypsin was set as the enzyme. A peptide mass tolerance of 8 p.p.m. and a fragment mass tolerance of 0.8 Da were allowed. Only peptides with high stringency Mascot Score were used for protein identification. Peptide false discovery rate<1% was used. For each pull-down experiment, three conditions were used to select specific proteins complexes from experimental contaminants: control beads without peptides, AmotL2Delta3 peptides lacking the three last amino acids, and the full-length-positive peptides. Only proteins that bound only to full-length AmotL2 peptides were shown in Supplementary Table 1. Tables showing whole experimental proteins list were enclosed in Supplementary Data 1 and 2 (CACO2_PullDown_AMOTL2_AMOTL2Del_CrtlBeads_WHOLEPROTEINLIST and HeLa_PullDown_AMOTL2_AMOTL2Del_CrtlBeads_WHOLEPROTEINLIST). Immunoprecipitation HeLa and Caco-2 cell lysates were immunoprecipitated with AmotL2 polyclonal antibodies (reactive to AmotL2 C-terminal peptide). Immunocomplexes bound to protein A sepharose beads were gently washed five times with lysis buffer (50 mM HEPES buffer, pH 7.4, 150 mM NaCl, 0.1% SDS, 1% Triton X-100, 1 mM EGTA and protease inhibitors) and separated by SDS-PAGE. Immunofluorescent staining Cells were cultured in eight-well chamber slides, fixed with 4% paraformaldehyde at room temperature and permeabilized in 0.1% Triton X-100. Nonspecific reactivity was blocked by pretreatment of slides with 5% horse serum in PBS. Primary antibody diluted in blocking buffer was incubated at room temperature for 1 h. The following commercial antibodies were used; Par3 (1:100, Millipore), Trappc9 (1:25, Genetex), p100 AmotL2, Trappc10 (1:100, 1:50, Santa Cruz Biotechnology), ZO1 (1:100, Invitrogen), Ezrin and β-catenin (1:100, 1:100, BD Biosciences), Crb3 for immunohistochemistry and E-cadherin (1:50, 1:100, Sigma), and CA9 (1:100, R&D Systems), anti-Rab11 (1:50, 47/Rab11, BD Transduction Laboratories), anti-Rab8 (1:50, 4/Rab8, BD Transduction Laboratories), anti-Rabaptin5 (1:25, C-20, Santa Cruz Biotechnology), anti-EEA1 (1:50, 1D4, Abnova), anti-gm130 (1:50, 35/gm130, BD Transduction Laboratories), anti-USO1 (1:50, Proteintech), anti-Rab1 (1:100, Sicgen), anti-COPgamma (1:50, Sigma), anti-Tgoln2 (1:100, Sigma), anti-LAMP1 (1:200, Abcam), anti-LAMP2A (1:100, Abcam), LysoTrackerRed DND-99 (75 nm, Life Technologies). Immunoaffinity-purified rabbit polyclonal antibodies against the C-terminal 20 amino acids of human AmotL2 was used in paraffin sections have been previously described (Hultin et al. ) [18] . For Amotl2, antibodies were also made against the epitope NH2- CQKAPSAVDLFKGVDDVSAE-COOH cross-reactive with human and zebrafish Amotl2. Positive staining was visualized using fluorescent-conjugated secondary antibodies (Molecular Probes). Images were captured by confocal microscope (Leica, TCS SP5). Images of Trappc9/10 and AmotL2 co-localization were processed with Imaris (Bitplane) to visualize overlapping signal. This was performed by creating a new co-localization channel, showing only the Trappc9/10-positive pixels that also were positive for AmotL2. Fluorescence recovery after photobleaching MDCK cells were seeded on glass bottom culture dishes (MatTek) at a density of 20,000 cells cm − 2 . Imaging was performed 20 h post transfection. RPMI without phenol red (Gibco) containing 10% fetal bovine serum and 1 mg l −1 Hoechst for DNA staining (Invitrogen) was used as recording medium. Time-lapse recordings were carried out with 350–500 frames of resolution of 512 × 512, 1,000 Hz and 2.218 s per frame using a confocal microscope (Leica TCS SP5). Hoechst, green fluorescent protein and Cherry were excited using 405, 488 and 543 nm lasers, respectively. Five frames were recorded pre-bleach. Bleaching was set to 1 s and 100% laser intensity using a tornado pattern with an Olympus FV1000 confocal microscope. Fluorescence resonance energy transfer p60 AmotL2 or p60ΔPDZ AmotL2 was overexpressed with a tetracycline inducible system in MDCK cells. Two days after induction of protein expression, cells were fixed with 4% paraformaldehyde, and permeabilized with 0.1% Triton X-100. Thereafter, cells were stained with anti-AmotL2 immunoaffinity-purified antibody labelled with Zenon Alexa488 Rabbit IgG labelling Kit (Life Technologies). Endogenous Par3 was stained with anti-Par3 rabbit polyclonal antibody (Millipore), which was labelled with anti-rabbit Cy3 (1:1,000, Life Technologies). For CellTrackerGreen (Life Technologies) loading, cells were incubated with the dye for 1 h at 37 °C, followed by incubation in fresh medium without dye for 30 min, before fixation and immunofluorescent staining. FRET recordings were performed using the FRET donor–acceptor pair Alexa488-Cy3 (ref. 50 ) FRET was detected by acceptor photobleaching in a region where the proteins were co-localized (1–2 μm 2 ) by continuous excitation with the 561 nm laser for 10–20 s. Thereafter, the residual Alexa488 and Cy3 signals were detected, with a Zeiss LSM5 Exciter, using using band-pass filter 505–530 nm and long-pass filter 575 nm. A region of interest was outlined in the photo-bleached area and processed using Zeiss LSM software. Ratios between the donor intensities (Alexa488) in the region of interest, before and after photobleaching, were calculated to quantify FRET. The FRET efficiency was calculated according to the formula E =1− D b / D d , where E is FRET efficiency, D b is the fluorescence intensity of donor before acceptor bleaching, and D d is the fluorescence intensity of donor after acceptor bleaching. The FRET values presented are corrected for erroneous intensity changes in an unbleached area and for bleaching of donor fluorochrome. Transient and stable transfection Plasmid constructs were transfected using Lipofectamine 2,000 according to the manufacturer’s protocol (Invitrogen). For establishing stable cell lines, 3 days after transient transfection, the corresponding antibiotics were added to the culture medium for selection at the following concentrations: 0.6 mg ml −1 G418 or together with 5 μg ml −1 blasticidin for stable transfected HeLa cells; and 1.0 mg ml −1 G418 or together with 5 μg ml −1 blasticidin for stable transfected MDCK and Caco-2 cells. Gene silencing via siRNA A pool of four distinct siRNA directed against the genes of interested was designed using a proprietary algorithm and commercially purchased (siGENOME Smartpool, Dharmacon Inc.). HeLa cells were transfected with human HIF-1α, HIF-2α or AmotL2 siRNA using oligofectamine transfection reagent (Invitrogen). siRNA scrambled controls were included as controls in all experiments. The efficiency of the gene silencing was examined by western blotting 72 h after siRNA transfection. Matrigel cyst formation assay Growth of cysts in 3D Matrigel (BD Biosciences) was performed as previously described [51] . A suspension of single cells with a concentration of 2 × 10 4 cells ml −1 was mixed 1:1 with diluted 4% Matrigel in order to give a final concentration of 2% Matrigel. Each well of an eight-well chamber slide was coated with 100% Matrigel and incubated at 37 °C for 5 min. For in vitro invasion assays, MDCK and Caco-2 cells were allowed to form cyst structures in 3D Matrigel. After 72 h culture, 1 μg ml −1 doxycycline (Sigma) was added to the culture media to induce p60 AmotL2 expression in the stable transfected MDCK and Caco-2 cells. Forty-eight hours after doxycycline treatment, 15 and 5 ng ml −1 HGF were added to the MDCK and Caco-2 culture media, respectively. Invasive cysts were visualized using phalloidin actin staining and scored 48 h after initiation of HGF stimulation. In vivo tumour growth Animal experiments were performed according to a permit from the Stockholm South ethical committee in Sweden. SCID mice of 6- to 8-week old were used for tumour injection. Approximately, 2 × 10 6 Caco-2 or AmotL2 stable transfected Caco-2 cells were mixed with 2 × 10 4 NIH3T3 cells and injected subcutaneously. Tumour development was monitored and tumour size was measured every other day with calipers. The tumour volumes were calculated by the formula 0.52 × length × width 2 . Sections with the thickness of 5 μm were cut from formalin-fixed, paraffin-embedded tumours and used for immunohistochemistry. 66C14 cells (5 × 10 5 ), labelled with luciferase and infected with Amotl2 shRNA or control vector, were injected into the fourth mammary fat pad of female Balb/C mice. The mice were monitored biweekly for tumour development by palpation, and fluorescence was measured by IVIS Xenogen Spectrum CT 15 min after intraperitoneal luciferin-D injection (150 mg kg −1 ). Mice were killed when the tumours reached a size of 10 mm 3 . Lentiviral production and infection Envelope vector pSPAX2, packaging vector pMD2.G and viral cloning vector pLKO.1-TRC as pLKO.1 scramble shRNA vector were purchased from Sigma-Aldrich. AmotL2 shRNA oligos targeting mouse AmotL2 mRNAs were cloned into the pLKO.1-TRC vector. The target sequence for the mouse AmotL2 knockdown construct was 5′-CAGTACCCACACGCTGTAATG-3′. Lentiviral particle were produced by transfecting HEK293T cells with the pMD2.G, the pSPAX2 and the pLKO.1-TRC cloning vector containing either the AmotL2 shRNA constructs or the scrambled shRNA constructs. Viral particle were collected after 48 h of transfection, supplemented with 8 μg ml −1 protamine sulphate and used to infect 66C14 mouse cells. Statistical analysis Data from at least three independent experiments are presented as mean±s.d. Comparisons between different groups were analysed for statistical significance with the Student’s unpaired t -test. A value of P <0.05 was considered as statistically significant. For mouse experiments, seven mice were assigned per group. This sample size gave 80% power to detect a 60% phenotypic difference with 95% confidence. For breast tumours from patients, at least 50 patients were included in each group. This sample size was calculated so that we would have 80% power to detect a difference of 30% between the groups with 95% confidence. For the colon samples, it was harder to obtain tumours of Dukes A stage compared with Dukes B–C or normal colon (ratio Dukes A/normal colon ~0.4). Hence, different number of samples was used in the different groups. A sample size of 14 and 35 patients for the different categories, respectively, allowed us to detect a difference of 50%, with 80% power and 95% confidence. How to cite this article: Mojallal, M. et al. AmotL2 disrupts apical–basal cell polarity and promotes tumour invasion. Nat. Commun. 5:4557 doi: 10.1038/ncomms5557 (2014).